A 520 million-year-old chelicerate larva An important survival strategy for animal species is the so-called niche differentiation between larva and adult. Different developmental stages of the same animal occupy different ecological niches to avoid competing for food or other essential resources. Here, we describe an exceptionally preserved larval stage of the short great appendage (SGA) arthropod (megacheiran) Leanchoilia illecebrosa from the early Cambrian Chengjiang biota of China. The larval specimen preserves fine details of the main feeding limb, the SGA, which are unknown in the adult of the same species. This discovery demonstrates that niche differentiation during ontogeny was developed in this species of megacheiran—a group of fossil arthropods that has been considered to be early representatives of Chelicerata, which includes horseshoe crabs and arachnids. Hence, this type of niche differentiation, which is common today, originated from the early Cambrian. Arthropods have dominated faunas from the early Cambrian (~520 million years ago) [1] to the present [2] . Being both abundant and diverse in the fossil record, arthropods provide a proxy for the early evolution of animals, as few other groups preserve similarly detailed fossil evidence. One of the survival strategies of arthropods is the so-called niche differentiation between larva and adult, which prevents the young from competing with their parents for food or other essential resources, and in turn, increases the survival rate of the species [3] , [4] . Such niche differentiation is based on morphological differences between larva and adult, as seen in the development of many extant arthropods [5] . An arthropod larva often possesses structures that are important for its mode of life but become reduced or lost during ontogeny. For example, the temporary sensory organs, the frontal filaments in the head of planktonic barnacle larvae, degenerate and are absent in the sessile adult [6] , [7] . Compared with extant arthropods, our knowledge of niche differentiation during ontogeny in fossil taxa remains poor, partly due to the difficulty of identifying morphological differences between larva and adult specimens. The short great appendage (SGA) arthropod—or megacheiran— Leanchoilia illecebrosa is one of the most abundant species from the ~520 million-year-old Cambrian Chengjiang biota, Yunnan province, southwest China [8] . The phylogenetic placement of megacheirans is controversial, but the position of the SGA on the first post-ocular segment has been homologized with that of the chelicera of extant chelicerates [9] , [10] , [11] , [12] supporting the assignment of megacheirans to Chelicerata sensu lato (=chelicerate total group; for other phylogenetic interpretations, see refs 13 , 14 , 15 ). It is in this sense [10] that we refer to megacheira as chelicerates here. As an early chelicerate, L. illecebrosa offers important insights into the early evolution of this major arthropod group. Most specimens of L. illecebrosa range in body length from 20 to 46 mm (ref. 16 ); specimens smaller than 20 mm are rare. 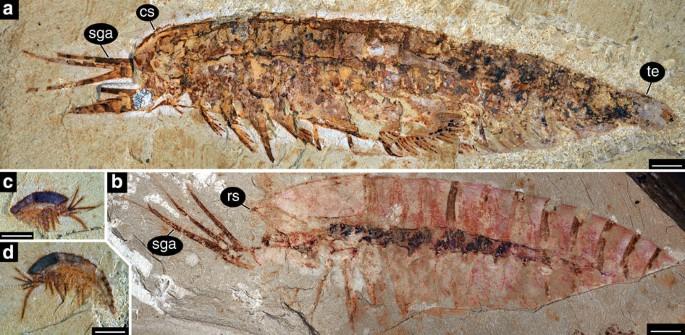Figure 1: Adult and larval specimens ofL. illecebrosa. (a) Dorsolateral view of adultL. illecebrosa(YKLP 11082); (b) lateral view of adultL. illecebrosa(YKLP 11083); (c,d) Part and counterpart of larvalL. illecebrosa(YKLP 11084a, b). cs, cephalic shield; sga, short great appendage; rs, rostrum; te, terminal end piece. Scale bars, 2 mm. Here, we report a specimen with a body just 8 mm long; only one of similar size is known (Figure 11a in ref. 17 ; specimen is currently not available for study). Our specimen represents a larval stage and preserves fine details of the SGA, which are unknown in the adult of the same species. This discovery suggests that niche differentiation during ontogeny originated by the early Cambrian. General morphology Body organized into head and trunk ( Fig. 1c,d ). The cephalic shield ( Fig. 2a ), with a short rostrum in the front, comprises four appendage-bearing segments. The eyes are not apparent. The trunk, like that of adult L. illecebrosa ( Fig. 1a,b ), comprises 11 segments followed by a dagger-shaped terminal end piece, presumably the telson. There is no evidence of post-embryonic segment addition in megacheirans such as L. illecebrosa (contra (ref. 17 ), their Figure 11). Figure 1: Adult and larval specimens of L. illecebrosa . ( a ) Dorsolateral view of adult L. illecebrosa (YKLP 11082); ( b ) lateral view of adult L. illecebrosa (YKLP 11083); ( c , d ) Part and counterpart of larval L. illecebrosa (YKLP 11084a, b). cs, cephalic shield; sga, short great appendage; rs, rostrum; te, terminal end piece. Scale bars, 2 mm. 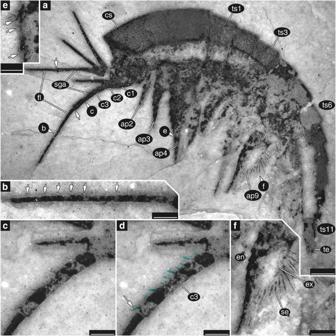Figure 2: Fine details of larval stage ofL. illecebrosa. (a) Counterpart (YKLP 11084b), incorporating information from the part (YKLP 11084a). Arrows mark articulation between third claw element of short great appendage and flagellum. Small letters with arrowheads point to areas of which close-ups were made. (b) Part, flagellum of distal claw element; arrows mark short setae arising disto-medially from each flagellomere. (c,d) Counterpart, distal claw element. At least ten setae (marked in cyan ind) arise from the median margin of the claw element 3 (c3). No distal hook-like spine (arrow) is present in contrast to the adult (Fig. 3a). (e) Counterpart, endopod of appendage 4; arrows mark setae. (f) Part, appendage 9 showing well-preserved endopod and exopod. Further abbreviations: ap, appendage; c, claw element, en, endopod; ex, exopod; fl, flagellum; ts, trunk segment. Scale bar: (a) 500 μm, (b–d) 200 μm, (e) 180 μm, (f) 300 μm. Full size image Figure 2: Fine details of larval stage of L. illecebrosa . ( a ) Counterpart (YKLP 11084b), incorporating information from the part (YKLP 11084a). Arrows mark articulation between third claw element of short great appendage and flagellum. Small letters with arrowheads point to areas of which close-ups were made. ( b ) Part, flagellum of distal claw element; arrows mark short setae arising disto-medially from each flagellomere. ( c , d ) Counterpart, distal claw element. At least ten setae (marked in cyan in d ) arise from the median margin of the claw element 3 (c3). No distal hook-like spine (arrow) is present in contrast to the adult ( Fig. 3a ). ( e ) Counterpart, endopod of appendage 4; arrows mark setae. ( f ) Part, appendage 9 showing well-preserved endopod and exopod. Further abbreviations: ap, appendage; c, claw element, en, endopod; ex, exopod; fl, flagellum; ts, trunk segment. Scale bar: ( a ) 500 μm, ( b – d ) 200 μm, ( e ) 180 μm, ( f ) 300 μm. Full size image SGA The first post-ocular head segment bears a pair of uniramous SGA with a basal peduncle and distal multichela (claw) [10] comprising two and three elements, respectively ( Fig. 2a ). The most distal finger (claw element 3) of the multichela carries a flagellum. Presumably the other fingers also had flagella, but these are not preserved (we cannot exclude the possibility that they only developed later in ontogeny, further differentiating larva and adult). Each of the articles of the preserved flagellum carries a short medio-distal seta ( Fig. 2b ). Claw element 3 is about 840 μm long and about 140 μm wide at the base, that is, about six times as long as wide ( Fig. 2c ). It bears a series of at least ten tiny spine-like armatures (<100 μm long) along its medial margin, about 50 μm apart ( Fig. 2c,d ). These armatures point medially to medio-distally; successively more distal examples make a progressively lower angle with the claw element. Biramous appendages Each trunk tergite is associated with a pair of biramous appendages similar to those posterior to the SGA in the head. They consist of a basipod, which carries an elongate endopod medio-distally and a paddle-shaped bipartite exopod latero-distally, the latter bearing around 14 long setae along its lateral and distal margins ( Fig. 2e,f ). We interpret the small specimen (YKLP 11084; Figs 1c,d and 2 ) described here as representative of L. illecebrosa based on: (i) the occurrence of associated adult specimens at the same locality; (ii) the overall morphology including the 11-segmented trunk and dagger-like terminal end piece; (iii) the morphology of the biramous appendages and (iv) the shape of the head shield with a pointed rostrum ( Table 1 ; see also ref. 11 ). Furthermore, we interpret the new tiny specimen as a larval stage of L. illecebrosa as it possesses structures that are no longer present in the adult, that is, the spine-like armature on the SGA. These structures are interpreted as lost during ontogeny, a common characteristic of larval stages. These morphological differences indicate that larva and adult occupy different ecological niches. The tiny individual differs from larger specimens of L. illecebrosa mainly in the morphology of the third claw element of the multichela ( Figs 3 and 4 ). This element has a length-to-width ratio of 6:1 in the larva, but 10:1 in the adult (length: 6.25 mm in YKLP 11083, at least 6.6 mm in YKLP 11082; width at base: 0.63 mm in YKLP 11083, 0.69 mm in YKLP 11082; Fig. 3a–d ; Table 1 ; similarly elongate elements are present in adults of other Leanchoilia species, see ref. 10 ). The width is constant in the larva but reduces distally in the adult. Most importantly, the tiny spine-like armatures that are present along the medial margin of the third claw element and its flagellum in the larva are absent in associated larger specimens of L. illecebrosa . Similar structures have not been observed in any other species of Leanchoilia except for a new undescribed form ref. 18 , in which the armature is different. The only armature known on the SGA of adult L. illecebrosa is the distal hook-like spine ( Figs 3 and 4 ), which presumably corresponds to the separate claw element 4 in other leanchoiliids [9] , [10] . This hook-like spine is absent in the larva but a longer seta inserts in the same position ( Fig. 2d ). The base of the flagellum in the larva is only slightly narrower than claw element 3 and arises axially ( Fig. 2c ). By contrast, the flagellum in the adult is much thinner than claw element 3 and arises laterally from this element ( Fig. 3a,b )—a feature shared by all other leanchoiliids, where it is known [10] . In sum, the differences between the tiny and large morphs of L. illecebrosa suggest a different autecology for larva and adult. Table 1 Comparison of larval and adult morphology of Leanchoilia illecebrosa. 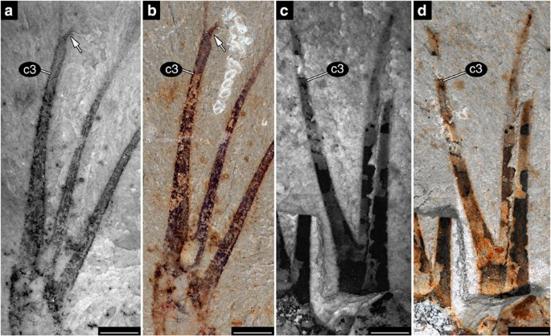Figure 3: Details of the SGA in adultL. illecebrosa. (a,b) Close-up of the SGA inFig. 1b. The spine-like armature observed on the SGA of the larva is absent here in the adult. The hook-like spine (arrow) of claw element 3 is elongate compared with that of the larva (Fig. 2c). (c,d) Close-up of the SGA inFig. 1a. The SGA of this adult specimen does not bear any spine-like armatures either (here distal part broken off, thus hook-like spine missing).aandcare composite-fluorescence images;banddwere photographed under cross-polarized light. Abbreviations as before. Scale bars, 1 mm. Full size table Figure 3: Details of the SGA in adult L. illecebrosa . ( a , b ) Close-up of the SGA in Fig. 1b . The spine-like armature observed on the SGA of the larva is absent here in the adult. The hook-like spine (arrow) of claw element 3 is elongate compared with that of the larva ( Fig. 2c ). ( c , d ) Close-up of the SGA in Fig. 1a . The SGA of this adult specimen does not bear any spine-like armatures either (here distal part broken off, thus hook-like spine missing). a and c are composite-fluorescence images; b and d were photographed under cross-polarized light. Abbreviations as before. Scale bars, 1 mm. 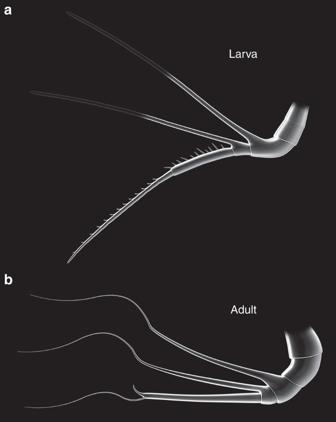Figure 4: Three-dimensional computer models of the SGA ofL. illecebrosa. (a) Larva. The flagella, supposedly present but not observed on the specimen, are shown fading out. (b) Adult. Not to scale. Full size image Figure 4: Three-dimensional computer models of the SGA of L. illecebrosa . ( a ) Larva. The flagella, supposedly present but not observed on the specimen, are shown fading out. ( b ) Adult. Not to scale. Full size image Extant arthropods have small cuticular sensory setae called sensilla that receive mechanical or chemical input from the environment [19] . The morphology of such sensilla is very similar in all arthropods: they are usually slender, delicate and always arise in a socket [19] . The spine-like armatures on the SGA of the L. illecebrosa larva, in contrast, are more robust and do not appear to articulate at the base. Although we cannot exclude a possible sensorial function for the armature, it seems more likely that these structures were involved in feeding. As this appendage was most likely used in grasping, it must have targeted different items than the adult. Given the separation between elements of the spine-like armature of about 50 μm, it may have trapped items down to this size, but at least objects in the sub-millimeter range. Such feeding may involve predation, but could include items such as foraminiferans or algae. It is not clear how food items were transported to the post-SGA appendages in either larva or adult [10] . The adult, in contrast to the larva, most likely caught significantly larger prey with the elongate distal claw element and the pronounced hook ( Fig. 4b ; see also ref. 16 ). Thus, this represents the first evidence of pronounced niche differentiation in a Cambrian megacheiran. The ontogeny of early crustaceans and even representatives of extant groups in the Cambrian is quite well known [20] , [21] , [22] , [23] , [24] , but evidence for larval stages of other arthropod groups remains rare. Even trilobite ontogenies are known only on the basis of the dorsal hard parts (refs 25 , 26 , 27 and references therein). Our knowledge of the ontogeny of other Cambrian megacheirans is limited to Yohoia tenuis from the Burgess Shale [28] . Specimens of Y. tenuis range in length from about 6 to 20 mm. Here too the number of body segments remains the same and the only significant morphological change is in the great appendage. In contrast to L. illecebrosa , the appendage becomes more robust during ontogeny. Thus, niche differentiation seems to have been less pronounced in Y. tenuis than in L. illecebrosa. However, the largest known stage in Y. tenuis is only about three times as large as the smallest, whereas the larger specimens of L. illecebrosa are more than 4.5 times the size of the larva. Hence, the difference between unknown earlier larval stages and adult Y. tenuis may have been greater. This preliminary evidence suggests that niche differentiation may have been greater between the larvae of megacheiran species than the adults. Thus, the ecological niches of the larvae differed not only from that of the adult but also from those of the larvae of closely related species. This interpretation emphasises that the Cambrian ecosystem already included species with complex life cycles and distinct niche differentiation. Material All investigated specimens of L. illecebrosa (YKLP 11082–11084) are housed at the Yunnan Key Laboratory for Palaeobiology, Yunnan University, Kunming, China. Locality and horizon All specimens were collected from the Yu’anshan Member of the Heilinpu Formation (Cambrian Series 2, Stage 3) at Ericaicun village, Haikou, Yunnan Province, China. Imaging Specimens were documented as a composite-fluorescence image with a Keyence BZ-9000 fluorescence microscope. A stack was recorded for each image detail and fused to a sharp image with CombineZM/ZP; all fused images were combined to a single high-resolution image with Microsoft Image Composite Editor or the Photomerge function of Adobe Photoshop CS3 (ref. 29 ). The specimen shows no fluorescence, in contrast to the surrounding matrix. Such inverse fluorescence is characteristic of Chengjiang fossils [28] . Part and counterpart were projected onto each other to achieve a composite view of all the morphological detail available. These specimens were documented as composite images under polarized light to enhance the contrast between specimen and matrix [30] . Reconstructions For the three-dimensional reconstructions in Fig. 4 the freely available software Blender was used. How to cite this article: Liu, Y. et al. A 520 million-year-old chelicerate larva. Nat. Commun. 5:4440 doi: 10.1038/ncomms5440 (2014).